Topological repulsion between domain walls in magnetic nanowires leading to the formation of bound states Head-to-head and tail-to-tail magnetic domain walls in nanowires behave as free magnetic monopoles carrying a single magnetic charge. Since adjacent walls always carry opposite charges, they attract one another. In most cases this long-range attractive interaction leads to annihilation of the two domain walls. Here, we show that, in some cases, a short-range repulsive interaction suppresses annihilation of the walls, even though the lowest energy state is without any domain walls. This repulsive interaction is a consequence of topological edge defects that have the same winding number. We show that the competition between the attractive and repulsive interactions leads to the formation of metastable bound states made up of two or more domain walls. We have created bound states formed from up to eight domain walls, corresponding to the magnetization winding up over four complete 360° rotations. The formation and manipulation of magnetic domain walls (DWs) is of considerable current interest both from a scientific and technological perspective. Technologically a number of very interesting and potentially useful memory [1] , [2] and logic [3] devices based on the controlled manipulation of DWs in magnetic nano-elements have recently been proposed and are under intensive investigation. Many of these devices depend critically on the detailed structure of the DW [4] , [5] . Since most studies to date have concentrated on individual DWs, there are very few reports on the interaction between DWs [6] , [7] , [8] , [9] . However, for many devices, the DWs must be closely packed and understanding their detailed short-range interaction is therefore critical. Head-to-head (HH) and tail-to-tail (TT) DWs are found in nanowires made of soft magnetic materials, in which the magnetization is constrained to align along the nanowire's length. These DWs are perhaps the simplest examples of movable magnetic monopoles [10] . They can be readily created in one-dimensional magnetic wires but this is more difficult in two- [11] and three-dimensional [12] magnetic systems. Since HH and TT walls carry opposite magnetic charges, they always attract one another when spaced further apart than their width. HH and TT DWs have complex structures [13] , [14] , typically vortex- (V) or transverse (T) wall structures, that can be described as composite objects composed of elementary topological defects [15] , [16] . These defects can be within the interior or at the edges of the nanowires. Interior defects have integer winding numbers, either +1 for a vortex or −1 for an anti-vortex, whereas edge defects have half-integer winding numbers, either +1/2 and −1/2. The DW net topological charge (including both interior and edge defects) is always zero, as discussed in ref. 16 . V walls are composed of one vortex and two edge defects, whereas T walls comprise two oppositely charged edge defects. The topological charges corresponding to V and T wall structures in a permalloy (Ni 81 Fe 19 ) nanowire are illustrated in Fig. 1a,b superposed on micromagnetic simulations of the respective magnetic configurations. 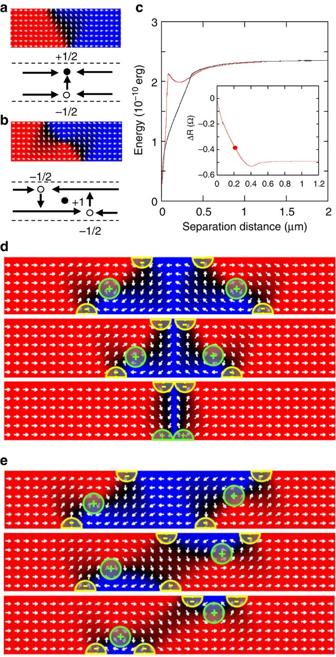Figure 1: Micromagnetic simulations of individual and interacting DWs. Simulations are performed for a 200 nm wide, 10 nm thick permalloy nanowire. Magnetization configurations for HH transverse (a) and vortex (b) walls. The local magnetization directions are indicated by arrows. The walls can be described in terms of interior and edge topological defects, as shown by the cartoons. (c) Energy calculated as a function of the separation distance for the two vortex walls with the same (red) or opposite (black) chirality. The inset shows the deviation of the nanowire's resistance from its value at saturation as a function of the separation distance for the two walls with opposite chiralities. The red dot shows the resistance for the distance corresponding to the bottom of the energy well. The magnetization profiles of vortex walls having the same (d) or opposite (e) chirality are shown for different separation distances. The position of the interior and edge topological charges are indicated by the + and − symbols. Figure 1: Micromagnetic simulations of individual and interacting DWs. Simulations are performed for a 200 nm wide, 10 nm thick permalloy nanowire. Magnetization configurations for HH transverse ( a ) and vortex ( b ) walls. The local magnetization directions are indicated by arrows. The walls can be described in terms of interior and edge topological defects, as shown by the cartoons. ( c ) Energy calculated as a function of the separation distance for the two vortex walls with the same (red) or opposite (black) chirality. The inset shows the deviation of the nanowire's resistance from its value at saturation as a function of the separation distance for the two walls with opposite chiralities. The red dot shows the resistance for the distance corresponding to the bottom of the energy well. The magnetization profiles of vortex walls having the same ( d ) or opposite ( e ) chirality are shown for different separation distances. The position of the interior and edge topological charges are indicated by the + and − symbols. Full size image Here we report a detailed study of the interactions between DWs in a permalloy nanowire. We show that, contrary to long-range interactions that are determined solely by the magnetic charges of the walls, short-range interactions are more subtle and depend on the detailed topological nature of the walls. We demonstrate that two vortex walls with the same chirality experience a strong repulsive interaction that suppresses their annihilation. The competition between this short-range repulsion and the long-range attractive interaction between the walls leads to the formation of bound states. We show that the bound states can be distinguished from the individual DWs themselves from the magnitude of their electrical resistance. Micromagnetic simulations of interacting DWs Micromagnetic simulations are used to calculate the energy of two V walls in a permalloy nanowire as a function of their separation distance d ( Fig. 1c ). The ground state of long permalloy nanowires is without any DWs. Thus, the presence of DWs always increases the energy of the nanowire. At large separations, the interaction energy is purely magnetostatic and is largely independent of the chiral character of the DWs. The energy is essentially determined by the magnetic charge of the DWs. When d is smaller than ~350 nm, the chiral nature of the DWs becomes important. When the two walls have opposite chiralities ( Fig. 1c , black line), their energy decreases monotonically at an increasingly faster rate as the two walls approach and annihilate each other. By contrast, for two walls of the same chirality ( Fig. 1c , red line), the energy reaches a local minimum at d ~250 nm and then increases for smaller d , before decreasing again as the two walls are annihilated. The existence of this energy minimum leads to the formation of a metastable DW bound state, whose properties are discussed below. We now discuss the origin of the repulsive interaction between the DWs in terms of their topological character. Fig. 1d,e compare the approach of two V walls of the same and opposite chirality, respectively, in a series of snapshots of the micromagnetic configurations as their separation decreases. The interior and edge topological defects are highlighted by green circles and yellow half-circles, respectively. When the approaching V walls have the same chirality, the closest edge defects between the two walls are along the same edge of the nanowire whereas, when the V walls have opposite chiralities, the closest edge defects are on opposite edges of the nanowire. In the latter case, as the two −1/2 edge defects from each of the approaching DWs along the same edge of the nanowire become closer, one of the two +1 interior defects approaches this edge and annihilates these two edge defects. This is possible because the combination of these three defects has zero net charge. This mechanism leads to ready annihilation of these V walls. By contrast, in the former case, two −1/2 edge defects approach each other along one edge of the nanowire without any intervening +1 interior defect so that these edge defects repel each other. This provides a significant energy barrier Δ E that prevents the annihilation of V DWs with the same chirality ( Fig. 1c ). When these two walls are forced towards one another, their vortex cores shift downwards and eventually annihilate at the bottom edge of the nanowire. This results in a 360° DW [17] , [18] , [19] , [20] with a net topological charge of zero, i.e., 2×−1/2 along the top edge and 2×+1/2 along the bottom edge. To estimate the magnitude of ΔE, it is useful to calculate the magnetic field needed to overcome this barrier. In the case shown in Fig. 1c , a field of ~+70 Oe is needed to overcome Δ E . This is a large value given that a negative field of the order of −100 Oe would be needed to overcome the attractive interaction between DWs of opposite chiralities separated by the same distance. In the metastable-bound state the distance between the DWs is much smaller than the individual width of isolated DWs. This means that the DWs are squeezed by their attractive interaction (second panel of Fig. 1d ). The extent of the compression can be quantified from the electrical resistance of the nanowire due to the anisotropic magnetoresistance (AMR) of permalloy. AMR has been demonstrated to be a very sensitive probe of the DW volume [5] . AMR leads to a slight decrease in resistance in the presence of DWs, because a portion of the magnetization in the DWs is oriented orthogonal to the current direction. The inset in Fig. 1c shows the resistance of the nanowire ΔR as a function of the distance between the DWs. (ΔR is calculated with respect to the nanowire resistance without DWs). When d is large, ΔR=ΔR 0 =−0.49 Ω, which is twice that for a single V wall, as expected for well separated DWs. When the DWs are closer, ΔR increases slightly as the walls start to interact with one another. However, the metastable-bound state (indicated by the solid circle in the inset to Fig. 1c ) corresponds to ΔR BS =−0.39 Ω, which is significantly smaller than ΔR 0 . The ratio ΔR BS /ΔR 0 indicates that the width of the bound state is ~72% of that of the two independent DWs. Bound states can also be formed with T walls [21] or a combination of V and T walls. Results from micromagnetic simulations are shown in Supplementary Figs S1 and S2 . Experimental demonstration of DW topological repulsion We now discuss experiments that demonstrate the topological repulsion between V DWs. Nano-devices are made from 6 μm long, 200 nm wide permalloy nanowires, to which metal contact lines are attached. The contact lines are used both to write DWs by generating large localized magnetic fields from current passed along one of the contact lines and to measure the nanowire resistance ( Fig. 2 ; Methods). As discussed above, the presence and number of DWs located in the nanowire between the electrical contacts can be deduced from the resistance of the nanowire. Moreover, the strength of the AMR signal also depends on the DW structure, whether V or T [5] . 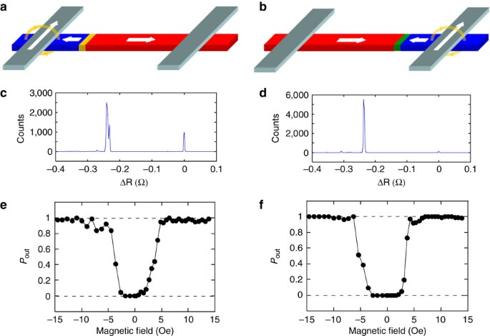Figure 2: Injection and motion of a single-domain wall. Data are measured in a 200 nm wide, 10 nm thick permalloy nanowire. The nanowire magnetization is first set rightward by a magnetic field (colour-coded in red), before tail-to-tail and head-to-head DWs are injected by passing a current pulse in the left (a) or in the right (b) contact lines (shown in grey), respectively. The direction of the current in the contact line (indicated by the white arrow) is such that the Oersted field (shown in yellow) switches the magnetization underneath the contact line leftward (colour-coded in blue). Resistance histograms shown in panels (c) and (d) are obtained by repeating this sequence many times. Panels (e) and (f) show the probabilityPoutthat the DW moves out of the nanowire when a magnetic field is applied along the nanowire. Figure 2: Injection and motion of a single-domain wall. Data are measured in a 200 nm wide, 10 nm thick permalloy nanowire. The nanowire magnetization is first set rightward by a magnetic field (colour-coded in red), before tail-to-tail and head-to-head DWs are injected by passing a current pulse in the left ( a ) or in the right ( b ) contact lines (shown in grey), respectively. The direction of the current in the contact line (indicated by the white arrow) is such that the Oersted field (shown in yellow) switches the magnetization underneath the contact line leftward (colour-coded in blue). Resistance histograms shown in panels ( c ) and ( d ) are obtained by repeating this sequence many times. Panels ( e ) and ( f ) show the probability P out that the DW moves out of the nanowire when a magnetic field is applied along the nanowire. Full size image Let us first consider the case in which a single domain wall is nucleated in the nanowire. Starting with the nanowire's magnetization fully saturated in the positive direction (rightward), a current pulse applied along the left contact line generates a TT wall at the left end of the nanowire ( Fig. 2a ). Similarly, a current pulse applied along the right contact line generates a HH wall ( Fig. 2b ). As shown by the histograms in Fig. 2c,d , the nanowire resistance is reduced by ΔR V =−0.24±0.01 Ω compared with its value at saturation. This value corresponds to the injection of a V wall. For a T wall, we find that ΔR T =−0.18±0.01 Ω in these nanowires. After the DW has been injected, a magnetic field is applied along the nanowire and the probability P out of the DW moving out of the nanowire is determined from changes in ΔR ( Fig. 2e,f for TT and HH DWs, respectively). When the magnetic field exceeds a threshold value of ~±5 Oe, the DW exits the nanowire with a high probability by moving either to the left or to the right, depending on its magnetic charge (HH or TT) and the field direction. These threshold values define the propagation field required to overcome pinning of the DWs in the nanowire likely due to edge and/or surface roughness. To probe their interaction, two DWs are nucleated from the same contact line (here the left contact) by applying two consecutive injection pulses with opposite polarities ( Fig. 3a ). We take advantage of our previous studies of current-driven DW motion in these nanowires [1] . We have shown that, owing to the spin transfer torque mechanism [22] , [23] , [24] , DWs can be moved along the nanowire over a distance controlled by the length of the injection pulse [7] , [25] (see Methods). Thus, when the first injection pulse is much longer than the second one, the two DWs are well separated, as shown in Fig. 3b for injection pulse lengths of 25 and 10 ns, respectively. In this case, the resistance histogram exhibits peaks at ΔR~−0.475 and ΔR~−0.415 Ω, very close to 2ΔR V and (ΔR V +ΔR T ), respectively. In both cases, the exit probability P out becomes distinctly asymmetric as a function of the magnetic field ( Fig. 3c,d ), contrary to the case of a single DW described above. For negative fields, the two walls are pulled away from one another. The propagation field is similar to that of a single wall, albeit slightly larger because of the long-range attractive interaction between the DWs. On the contrary, for positive fields, the two walls are driven towards one another until they collide. Thus, the threshold field above which P out approaches 1 indicates annihilation of the two walls rather than propagation towards the opposite ends of the nanowire. In many cases—~70% for two V walls and ~50% for one T wall and one V wall, respectively—the two DWs are annihilated in a field of ~5 Oe, which is very similar to the propagation field of a single DW. The walls annihilate as soon as the field is sufficient to cause them to move. By contrast, in the remaining cases, the magnetic field must exceed much larger fields of ~60 Oe to annihilate the DWs. This clearly shows that there is a strong repulsive force between the walls that must be overcome to annihilate them. 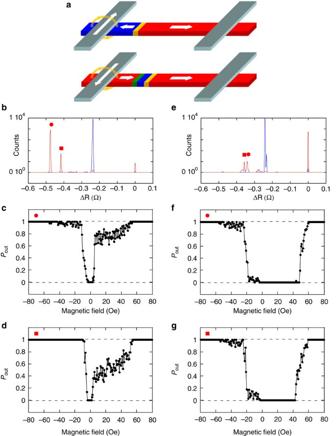Figure 3: Formation of bound states by injection of two DWs. (a) The two DWs are injected successively at the left contact line by reversing the injection pulse polarity. (b) The histograms after the first and second injection pulses are shown by the blue and red solid lines, respectively. The first and second injection pulse lengths are 25 and 10 ns, respectively. (c,d) show the probabilityPoutthat the DWs move out of the nanowire or annihilate when a magnetic field is applied along the nanowire. (c,d) correspond to the two peaks in the histogram shown in (b), as indicated by the symbols. Results obtained when both injection pulses are 10 ns long are shown in panels (e–g). Figure 3: Formation of bound states by injection of two DWs. ( a ) The two DWs are injected successively at the left contact line by reversing the injection pulse polarity. ( b ) The histograms after the first and second injection pulses are shown by the blue and red solid lines, respectively. The first and second injection pulse lengths are 25 and 10 ns, respectively. ( c , d ) show the probability P out that the DWs move out of the nanowire or annihilate when a magnetic field is applied along the nanowire. ( c , d ) correspond to the two peaks in the histogram shown in ( b ), as indicated by the symbols. Results obtained when both injection pulses are 10 ns long are shown in panels ( e–g ). Full size image To probe the range of this repulsive interaction and to determine whether bound states can indeed be formed, we reduce the separation distance between the two DWs by shortening the injection pulse length for the first DW ( Fig. 3e–g ). In this case, the resistance histogram after the second injection pulse exhibits a large peak at ΔR=0, indicating that the two DWs annihilate as soon as the second wall is injected ( Fig. 3e ). This annihilation occurs with a probability of ~45%. The histogram also exhibits two peaks at ΔR ~−0.34 and −0.36 Ω, and a weaker broad peak centred on ΔR~−0.28 Ω, none of which correspond to any combination of two independent V or T walls. These peaks correspond to intermediate values of resistance, suggesting the formation of bound states. This conclusion is also supported by the field dependence of P out ( Fig. 3f,g ). For positive fields, annihilation occurs at ~60 Oe, in good agreement with the previous data. However, contrary to these previous data, no annihilation occurs at low fields, because this already took place during the injection of the second wall ( Fig. 3e ). The negative field needed to pull the two DWs apart is ~20 Oe, more than 4 times the propagation field of an isolated vortex wall. This shows that the walls experience a strong attractive interaction, presumably, because they are very close to each other in this case. Control of the formation of bound DW states The formation of bound states can be controlled by varying the length of the two injection pulses t p 1 and t p 2 as shown in Fig. 4 . The probability of finding no DW, a single V DW, two independent V DWs, or a bound state is determined from the nanowire resistance, as measured after the first (top row) and second (bottom row) injection pulses. 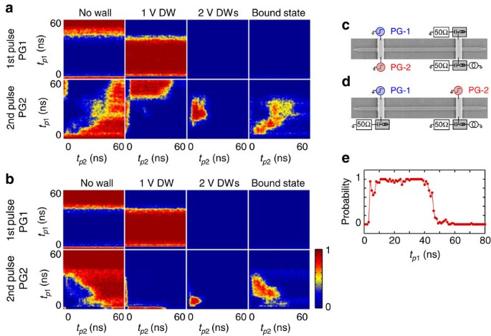Figure 4: Conditions under which bound DW states are formed. Colour maps of the probability of finding no wall, 1 V wall, 2 V walls or one bound state as a function of the length of the two injection pulses. The top and bottom rows show results obtained after the first and second injection pulses, respectively. (a,b) show results obtained when the DWs are injected from the same or opposite ends of the nanowire, respectively. Colour maps are created by binning data according to the resistance of the device (No wall: ΔR >−0.02 Ω, 1 V wall: ΔR=−0.24±0.01 Ω, 2 V walls: ΔR=−0.48±0.02 Ω, Bound state: −0.46<ΔR<−0.25 Ω). The electrical circuits used to inject DWs from the same end or opposite ends of the nanowire are shown schematically in (c,d), respectively. The probability of finding 1 V wall in the nanowire after the first injection pulse is shown in (e) as a function oftp1. Figure 4a,b shows data taken when the two DWs are injected from the same and opposite ends of the nanowire, respectively. The electrical circuits used in each case are shown in Fig. 4c,d . As discussed above, nucleation of a DW is followed by current-driven propagation of the DW along the nanowire by spin transfer torque. The longer the injection pulse, the farther away from the contact does the DW propagate. Indeed, for t p 1 >40 ns, the wall travels the full length of the nanowire during the first injection pulse, such that the probability of finding a single V wall decreases to zero (top two left probability maps in Fig. 4a,b,e ). During the second injection pulse, the two walls travel in the same direction due to spin torque, whereas dipolar interactions and Oersted field from the injection current favour attraction of the first injected wall towards the second one. Let us first discuss the case when the two DWs are injected from the same end of the nanowire ( Fig. 4a ). If the first injection pulse is longer than the second, the first DW travels far enough from the injection line, such that when the second DW is injected, the distance between the two DWs remains sufficiently large for them not to form a bound state but rather remain well separated. By contrast, when the length of the second injection pulse is similar to that of the first pulse and shorter than ~40 ns, a bound state can be formed with a high probability. When the second pulse is longer than ~40 ns, the two walls annihilate or are both shifted out of the nanowire. When the DWs are injected from opposite ends of the nanowire ( Fig. 4b ), the conditions of formation of the bound state are modified. The first injection pulse drives the first DW closer to the second injection line so that, contrary to the previous case, bound states are formed when the first injection pulse is longer than the second. The two DWs remain well separated when both injection pulses are shorter than ~15 ns, such that the DWs don't move far from the injection lines. Figure 4: Conditions under which bound DW states are formed. Colour maps of the probability of finding no wall, 1 V wall, 2 V walls or one bound state as a function of the length of the two injection pulses. The top and bottom rows show results obtained after the first and second injection pulses, respectively. ( a , b ) show results obtained when the DWs are injected from the same or opposite ends of the nanowire, respectively. Colour maps are created by binning data according to the resistance of the device (No wall: ΔR >−0.02 Ω, 1 V wall: ΔR=−0.24±0.01 Ω, 2 V walls: ΔR=−0.48±0.02 Ω, Bound state: −0.46<ΔR<−0.25 Ω). The electrical circuits used to inject DWs from the same end or opposite ends of the nanowire are shown schematically in ( c , d ), respectively. The probability of finding 1 V wall in the nanowire after the first injection pulse is shown in ( e ) as a function of t p 1 . Full size image We now compare the resistance levels of the bound states found experimentally to those derived from micromagnetic simulations. ΔR is directly proportional to both the AMR and resistivity of the nanowire, which can be deduced from the measured values for isolated V and T DWs. Using these values, we find that the resistance of bound states composed of two V walls, one V and one T DW, and two T DWs, are ΔR 2VB ~−0.35, ΔR VTB =−0.30, and ΔR 2TB =−0.24 Ω, respectively. The two peaks found experimentally at −0.34 and −0.36 Ω in Fig. 3e are very close to the calculated value for bound V walls, whereas the peak at −0.28 Ω is consistent with a combination of a V and a T wall. The existence of two peaks close to that calculated for the V bound state suggests the formation of two slightly different V bound states. We attribute this to local pinning effects, which can change the local potential energy landscape and thus stabilize bound states with different core-to-core distances. We find that the resistance level of a bound state can be changed slightly when a magnetic field smaller than the threshold values for annihilation or propagation is applied ( Supplementary Fig. S3 ). Presumably the bound state can be stretched or compressed depending on the direction of the applied field. A fine structure can also be observed in the resistance of single walls probably because of slight modifications of the DW width due to variations of the local pinning ( Fig. 2c ; Supplementary Fig. S4 ). When a bound state is formed, the nanowire's magnetization winds up by 360° across the bound state. To explore whether the magnetization can be wound up further, we apply up to 8 consecutive injection pulses. Examples of the resistance levels after each of the injection pulses are shown in Fig. 5 . In most cases, pair-wise DW annihilation is clearly evidenced by an increase of ΔR after each even injection pulse ( Fig. 5a,b ). However, in some other cases, the resistance decreases monotonically, showing that no annihilation takes place and that 8 DWs are indeed positioned in the nanowire after the 8 injection pulses ( Fig. 5c,d ). Interestingly, in the example shown in Fig. 5d , the resistance levels are consistent with the pairwise formation of four independent bound states; for odd injection pulses, the resistance is reduced by ΔR V , indicating that one V wall is injected in the nanowire. By contrast, for even injection pulses, ΔR is reduced by a much smaller amount, indicating the formation of bound states with resistance levels corresponding to [ΔR VTB +ΔR 2VB +ΔR 2VB +ΔR VTB ]. This suggests that once formed, the bound states interact weakly with one another. In our previous work, we have shown that the typical separation distance necessary for neighbouring walls to remain stable without collapsing against one another during injection was about 2.5 μm (ref. 7 ). Thus, a nanowire would have to be more than 20 μm long for 8 independent walls to remain stable. Owing to the formation of bound states, much smaller separation distances are possible, such that these 8 walls are stable in a 6 μm long nanowire. Two possible configurations of 8 bound V walls calculated by micromagnetic simulations are shown in Fig. 5e,f . The resistance levels are ΔR=−1.57 and −1.65 Ω, respectively, in good agreement with the experimental data. The configuration corresponding to the data of Fig. 5d is shown in Fig. 5g . 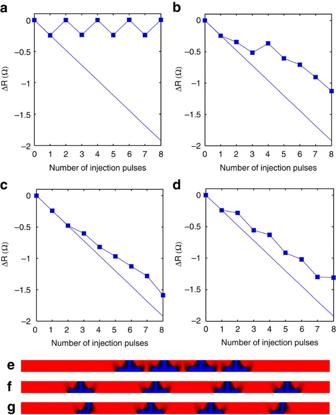Figure 5: Formation of bound states from eight DWs. (a–d) Examples of resistance levels measured after eight consecutive injection pulses, are applied. The solid blue line shows the values expected for 1 to 8 independent vortex walls. (e–g) Possible magnetization configurations of 8 DWs located in a 5 μm long, 200 nm wide, 10 nm thick permalloy nanowire, calculated by micromagnetic simulations. Figure 5: Formation of bound states from eight DWs. ( a–d ) Examples of resistance levels measured after eight consecutive injection pulses, are applied. The solid blue line shows the values expected for 1 to 8 independent vortex walls. ( e–g ) Possible magnetization configurations of 8 DWs located in a 5 μm long, 200 nm wide, 10 nm thick permalloy nanowire, calculated by micromagnetic simulations. Full size image In summary, we have shown that the topological repulsion between DWs with opposite magnetic charge leads to the formation of bound DW states. As these bound states interact weakly with one another, they can be packed much more closely along the nanowire than would otherwise be possible, thereby enabling denser DW-based devices. Micromagnetic simulations Micromagnetic simulations are performed using the LLG Micromagnetics Simulator software ( http://llgmicro.home.mindspring.com/ ). One HH and one TT DWs are generated at a distance of ~2 μm in a 4 μm long, 200-nm wide and 10-nm thick nanowire. The cell size is 5 nm×5 nm×10 nm. Periodic boundary conditions are applied along the nanowire length to cancel the demagnetizing fields due to the finite length of the nanowire. A magnetic field is applied to move the walls towards one another. The Zeeman energy from this driving field is subtracted from the total energy, so as to consider only the walls' internal energy and their interaction energy. The Gilbert damping constant is set to α =1 to minimize the contributions of the kinetic energy of the DWs due to their deformation. The centre-to-centre distance d between the walls is calculated from the net magnetization along the nanowire direction m x : d =(1− m x ) L /2 where L is the length of the nanowire. m x = M x / M S is the reduced magnetization (Ms=800 emu cm −3 for permalloy). Besides their chiralities, V walls are also characterized by the polarity of the vortex core, which has an important role in the dynamical behaviour of V walls. We find that the interaction energy is weakly sensitive to the polarity of the vortex cores of two approaching V walls. However, the interaction energy is slightly increased when the two vortices have the same polarity compared with when they have opposite polarities. The fields H an required to annihilate the bound states and H pull needed to pull the two walls away from one another are calculated directly from the energy profiles. For two V walls with the same chirality H an =70 Oe and H pull =−30 Oe. For one V wall and one T wall ( Supplementary Fig. S1a ), H an =55 Oe and H pull =−45 Oe. Finally, for two T walls ( Supplementary Fig. S1b ), we find that H an =110 Oe and H pull =−130 Oe. The increased value of H pull for bound states with T walls is a consequence of the smaller width of the T wall, which leads to narrower bound states and thus to stronger attractive interactions. The AMR signal is calculated from the DW structure by assuming the current flows homogeneously along the nanowire. This approximation is justified because the AMR in permalloy results in only a few percent change in resistivity. For a given magnetic structure, the decrease in resistance from that at saturation, ΔR, is proportional to the product of the resistivity ρ and the AMR ratio Δ ρ / ρ . To compare the simulated values with our experimental results, we scale the value obtained for a single DW, such that it matches the experimental value of ΔR V =−0.24±0.01 Ω. The scaling factor is ρ (Δ ρ / ρ )=0.337 μΩ.cm, which agrees well with the values measured experimentally in these nanowires ( ρ ~20 μΩ.cm, δ ρ / ρ ~1.5%). To check the validity of this scaling we compare the experimental value for a single T wall, ΔR T =−0.18±0.01 Ω with the calculated value and find excellent agreement. Device fabrication and experimental procedure Devices are fabricated by electron-beam lithography and argon-ion milling from a 10 nm thick permalloy film deposited by magnetron sputtering. The permalloy nanowires are straight lines, 200 nm wide and 6 μm long, terminated by pointed ends. A lift-off process is used to fabricate the two electrical contact lines that are made from 3 nm Ta/65 nm Rh. DWs are nucleated by the Oersted field from current pulses generated in the contact lines when the current exceeds a threshold of about 30 mA. The pulse voltage can be adjusted to favour one particular DW structure (either vortex or transverse). In this work, we use pulse voltages of −3.2V (corresponding to a current of ~45 mA) for which vortex walls are nucleated with a high probability. When an injection pulse is applied along one of the contact lines, a significant amount of the current also flows to ground through the nanowire. For the injection voltage used in this study, the current density in the nanowire is larger than the threshold for current-driven motion by spin-transfer torque. The current flowing through the nanowire has an important role in our experiments. Depending on its direction, it can drive the injected DW away from the contact line, or on the contrary, push it back towards the contact line and prevent nucleation. The electrical circuits and injection voltage polarities are chosen such that the DWs nucleated at the contact lines are pushed along the nanowire away from these lines by spin transfer torque. How to cite this article: Thomas, L. et al . Topological repulsion between domain walls in magnetic nanowires leading to the formation of bound states. Nat. Commun. 3:810 doi: 10.1038/ncomms1808 (2012).